The GOLD domain-containing protein TMED7 inhibits TLR4 signalling from the endosome upon LPS stimulation Toll-like receptor 4 is an innate immune receptor responsible for the recognition of the Gram-negative cell wall component lipopolysaccharide. Here we show that transmembrane emp24 domain-containing protein 7 (TMED7) inhibits MyD88-independent toll-like receptor 4 signalling. TMED7 overexpression inhibits the ability of TRAM, an adaptor utilized by toll-like receptor 4, or lipopolysaccharide to activate the interferon regulatory factor 3-signalling pathway, whereas TMED7 knockdown enhances production of the cytokine, RANTES, following lipopolysaccharide stimulation. Upon lipopolysaccharide stimulation, TMED7 co-localizes with TRAM and toll-like receptor 4 in late endosomes where it encounters the negative regulator of TRAM, TAG. The TMED7 sequence is found in TAG because of a read-through from the tmed7 gene into the ticam2 gene. TMED7 is essential for TAG-mediated disruption of the TRAM/TRIF complex and the degradation of toll-like receptor 4. A TMED homologue, logjam, has a negative role in the Toll and IMD pathways in Drosophila melanogaster ; therefore, TMEDs may have a conserved role in the regulation of innate immunity. Toll-like receptors (TLRs) are type 1 transmembrane receptors involved in the detection of invading pathogens. They possess a ligand-binding domain of leucine-rich repeats and a signalling Toll-IL-1 receptor (TIR) domain, which interacts with TIR domain containing adaptor molecules. TLR4 senses lipopolysaccharide (LPS) from Gram-negative bacteria [1] and launches a complex immune response. TLR4 is also reported to sense endogenous molecules produced during tissue injury, provoking inflammation [2] , [3] . Excessive host responses towards LPS have been shown to contribute to such diseases as Gram-negative sepsis, rheumatoid arthritis and atherosclerosis [4] . It is therefore essential that LPS-induced responses are tightly regulated. TLR4 activates two separate signalling pathways, the MyD88-dependent and MyD88-independent pathways. The TIR-domain containing adaptors Mal and MyD88 facilitate the activation of the MyD88-dependent pathway at the plasma membrane, resulting in the activation of the pro-inflammatory transcription factor nuclear factor (NF)-κB. TIR-domain-containing adaptor-inducing interferon-β (TRIF) and TRIF-related adaptor molecule (TRAM) facilitate the MyD88-independent pathway, leading to interferon regulatory factor 3 (IRF3) activation, which induces the expression of genes containing the interferon-sensitive response element (ISRE) in their promoter, such as those encoding interferon β (IFN β) and CCL5 (RANTES) [5] . Recent studies have revealed an important role for intracellular trafficking in the TLR ligand recognition and in the regulation of their downstream signalling pathways. Wang et al . [6] revealed that Rab10 acts as a positive regulator of TLR4 signalling by promoting transport of TLR4 from the Golgi to the plasma membrane. TLR4 and TRAM traffic from the plasma membrane to the early endosome upon LPS stimulation, and it is from these endosomes that the MyD88-independent pathway signals [7] . Rab7b acts as a negative regulator of the TLR4 signalling pathway by promoting the movement of TLR4 into late endosomes for degradation [8] , [9] , [10] . Husebye et al . [11] showed that Rab11a is essential for the trafficking of TLR4 into the Rab11a+ endocytic recycling compartment (ERC) and onto Escherichia coli -containing phagosomes. Rab11a knockdown reduced IRF3 signalling following E. coli (or LPS) stimulation, with little or no effect on NF-κB signalling. The transmembrane emp24 domain-containing protein (TMED)/p24 family are involved in the vesicular trafficking of proteins and are therefore functionally similar to the Rab family. Ten TMED genes are present in mammals and they are separated into four different subfamilies, α, β, δ and γ [12] . TMED proteins are highly conserved in eukaryotes [13] and exist as monomers, dimers, oligomers and hetero-oligomers [14] , [15] . They possess a GOLD domain, which is a β-strand-rich domain found in several proteins involved in Golgi dynamics, as well as intracellular protein trafficking [14] , [16] . Here we report on a TMED family member, TMED7, which negatively regulates TLR4 signalling. We have previously reported that the TMED7 transcript occurs in a protein we named TRAM adaptor molecule with GOLD domain (TAG), owing to a read-through from the gene encoding tmed7 into the ticam2 gene on chromosome 5 [9] , [17] , [18] . We now report that TMED7, like TAG [9] , acts as an inhibitor of the MyD88-independent TLR4 signalling pathway. TMED7 resides mainly in the Golgi and endosomal structures in resting cells. It co-localizes with TRAM intracellularly, but not TLR4, and is not present on the plasma membrane. Upon LPS stimulation, TMED7 trafficks into the maturing endosomal network along with TRAM and TLR4. Its GOLD domain appears to project into the cytosol where it can interact with TRAM and TAG, providing an explanation for why TAG has TMED7 in its sequence allowing for a homotypic interaction between the GOLD domains of TAG and TMED7. We have found that the disruption of the TRIF/TRAM complex by TAG requires TMED7, and that TMED7 targets TLR4 for degradation, resulting in the consequent cessation of TLR4 signalling. Our study therefore reveals a role for TMED7, as a critical inhibitor of TLR4 signalling, and implicates the TMED family, alongside the Rab family, as important regulators in the control of innate immune signalling. Expression profile of TMED7 It was originally reported that Tmed7 and Ticam2 ( Tram ) were two separate genes on chromosome 5; however, bioinformatics and experimental data have shown that there is a read-through from the Tmed7 gene into the Ticam2 gene, and this results in the expression of three genes, TMED7 , TRAM and TAG [9] , [18] . 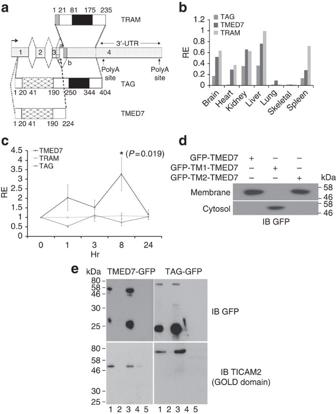Figure 1: Splicing and expression of TMED7 and TRAM, and TAG. (a) TMED7, TRAM and TAG are generated from alternative splicing of thetmed7-ticam2gene. The numbered grey boxes denote exons 1–4. The open reading frame for TRAM is read from exon 4 at the point marked 'a'. TAG mRNA is read from exons 1, 2, 3 and an alternative downstream splice acceptor site marked 'b' in exon 4. TMED7 mRNA is read from exon 1, 2 and 3 with an alternative splice site in exon 3 marked 'c'. Above the exons is a schematic representation of the TRAM protein, with its TIR domain (black box) and unique sequence containing the myristoylation site (dark grey box). Directly below the exons is a schematic representation of the TAG protein with its GOLD domain (hatched) and TIR domain (black). Below TAG is a schematic representation of the TMED7 protein with its GOLD domain (hatched). The boundaries of each domain are numbered according to their amino acid position. (b) An expression profile, generated by reverse transcription—PCR (RT–PCR), on a panel of human adult tissue using primers specific for TMED7, TRAM and TAG. Expression was normalized toGAPDHand is represented as a fold change relative to the amount ofTRAMexpressed in liver. Data are representative of one experiment performed with triplicate samples. (c) TMED7, TAG and TRAM mRNA levels were measured using quantitative RT–PCR in monocytes untreated and stimulated with LPS (100 ng ml−1). Expression was normalized toGAPDHand is presented relative to untreated cells. Data are representative of three experiments performed with triplicate samples and presented as mean ± s.d. The asterisk indicates statistical significance (two-tailed Student'st-test) ofP<0.05. (d) A membrane fractionation assay on HEK293 cells transfected with wild-type TMED7-GFP or TMED7 with the N terminus transmembrane mutated (GFP-TM1 TMED7) or with the C terminus transmembrane mutated (GFP-TM2 TMED7). (e) A biochemical protease protection assay of HEK293 cells expressing TMED7-GFP or TAG-GFP. Lane 1, WCL; lane 2, cytosolic fraction; lane 3, membrane fraction (MF); lane 4, MF plus trypsin; lane 5, MF plus trypsin plus Triton X100. The immunoblotting antibodies (IB) are listed beside the appropriate blot. Data are representative of three experiments. Figure 1a demonstrates how TMED7, TRAM and TAG are generated. TMED7 is a 224 amino acid protein containing the GOLD domain of TAG, but no TIR domain, plus a putative coil–coil domain. TMED7 has two putative transmembrane domains, one near its N terminus (aa 17–34) and another near its C terminus (aa 186–207). TMED7 and TRAM share no sequence identity. We analysed the TMED7, TAG and TRAM mRNA expression profile by quantitative PCR using a human multiple-tissue cDNA panel ( Fig. 1b ). The TMED7 expression profile was very similar to that of TRAM and TAG. The levels of TRAM were usually higher than TMED7, whereas the TAG expression levels were always lower. TMED7, TAG and TRAM were detected in all tissues with the highest expression found in liver and the lowest in skeletal muscle. We examined TRAM, TAG and TMED7 expression in monocytes, dendritic cells and macrophages, and found that in all three immune cell types, TRAM had the highest expression level, whereas TAG had the lowest expression level ( Supplementary Fig. S1 ). We investigated the levels of TMED7, TAG and TRAM mRNA expression upon LPS stimulation in human monocytes ( Fig. 1c ). Unlike TRAM, whose levels remain constant following LPS stimulation, TMED7 mRNA levels appear to increase upon LPS stimulation, peaking 1 h post-LPS stimulation. The levels then drop back down to basal levels by 3 h. A consistent and statistically significant second increase in TMED7 mRNA occurs at approximately 8 h with the levels returning to base line at 24 h. The role of this biphasic increase in TMED7 is presently unknown. A similar pattern of expression of TMED7 was observed at the protein level ( Supplementary Fig. S1 ). The biphasic increase appeared to be unique to LPS as the TLR ligands PolyI:C (TLR3) and CpG (TLR9) had no effect on TMED7 mRNA or protein levels ( Supplementary Fig. S1 ). To further characterize TMED7, we investigated the exact localization of the GOLD domain of TMED7. TMED7 possesses two potential transmembrane motifs (TM), one at the N terminus (aa 17–34, termed TM1), which is also present in TAG, and another at the C terminus (aa 186–207, termed TM2). To confirm if one or both of these potential TMs span the membrane, we used TMED7-green fluorescent protein (GFP) with the GFP tag at the C-terminus. The potential TMs at the N terminus (TM1) and C terminus (TM2) were individually mutated. A membrane fractionation assay demonstrated that the TM1 mutant resided exclusively in the cytosol, whereas the TM2 mutant still resides in the membrane ( Fig. 1d ). This demonstrated that TM1 is essential for TMED7 to span the membrane. We wished to determine if the GOLD domains of TMED7 and TAG reside in the lumen of the Golgi or project into the cytosol. A biochemical protease protection assay [19] revealed that the C-terminus GFP tag on TMED7 and TAG are sensitive to trypsin digestion in digitonin-permeabilized cells, suggesting that the C-terminus of TMED7 and TAG project into the cytosol ( Fig. 1e ). Using an antibody specific for the GOLD domain of TMED7 and TAG, we revealed that the GOLD domains of both of these proteins are also sensitive to trypsin digestion ( Fig. 1e ), suggesting that the GOLD domains protrude into the cytosol. This would allow the GOLD domains of TMED7 and TAG to interact in the cytosol where the TLR4/TRAM/TRIF complex occurs. Figure 1: Splicing and expression of TMED7 and TRAM, and TAG. ( a ) TMED7, TRAM and TAG are generated from alternative splicing of the tmed7-ticam2 gene. The numbered grey boxes denote exons 1–4. The open reading frame for TRAM is read from exon 4 at the point marked 'a'. TAG mRNA is read from exons 1, 2, 3 and an alternative downstream splice acceptor site marked 'b' in exon 4. TMED7 mRNA is read from exon 1, 2 and 3 with an alternative splice site in exon 3 marked 'c'. Above the exons is a schematic representation of the TRAM protein, with its TIR domain (black box) and unique sequence containing the myristoylation site (dark grey box). Directly below the exons is a schematic representation of the TAG protein with its GOLD domain (hatched) and TIR domain (black). Below TAG is a schematic representation of the TMED7 protein with its GOLD domain (hatched). The boundaries of each domain are numbered according to their amino acid position. ( b ) An expression profile, generated by reverse transcription—PCR (RT–PCR), on a panel of human adult tissue using primers specific for TMED7, TRAM and TAG. Expression was normalized to GAPDH and is represented as a fold change relative to the amount of TRAM expressed in liver. Data are representative of one experiment performed with triplicate samples. ( c ) TMED7, TAG and TRAM mRNA levels were measured using quantitative RT–PCR in monocytes untreated and stimulated with LPS (100 ng ml −1 ). Expression was normalized to GAPDH and is presented relative to untreated cells. Data are representative of three experiments performed with triplicate samples and presented as mean ± s.d. The asterisk indicates statistical significance (two-tailed Student's t -test) of P <0.05. ( d ) A membrane fractionation assay on HEK293 cells transfected with wild-type TMED7-GFP or TMED7 with the N terminus transmembrane mutated (GFP-TM1 TMED7) or with the C terminus transmembrane mutated (GFP-TM2 TMED7). ( e ) A biochemical protease protection assay of HEK293 cells expressing TMED7-GFP or TAG-GFP. Lane 1, WCL; lane 2, cytosolic fraction; lane 3, membrane fraction (MF); lane 4, MF plus trypsin; lane 5, MF plus trypsin plus Triton X100. The immunoblotting antibodies (IB) are listed beside the appropriate blot. Data are representative of three experiments. Full size image The location of TMED7 changes upon LPS stimulation Live-cell imaging was used to determine the location of TMED7, using TMED7 fused to CFP (TMED7-CFP), or GFP (TMED7-GFP). TMED7 appears to locate differentially to TRAM, which appears in the plasma membrane and in intracellular endosomal structures ( Fig. 2a ), and to TAG, which forms a reticular pattern throughout the cell ( Fig. 2a ). TMED7 has a thread-like perinuclear appearance in the cytosol ( Fig. 2a , white arrow), as well as appearing in small endosome-like structures ( Fig. 2a , orange arrow). GOLD domain containing proteins have been shown to be involved in bidirectional transport at the endoplasmic reticulum (ER)–Golgi interface. We investigated whether TMED7 could, like TAG, locate to the ER. Although there is some co-localization between the ER and TMED7 basally ( Supplementary Fig. S2 ), further investigation revealed that TMED7 resides mainly in the Golgi ( Fig. 2b ). Considering that TMED7 expression appears to be regulated by LPS, we next investigated whether TMED7 location was, like TRAM and TAG, affected by LPS stimulation. TMED7 localized to a Golgi-like perinuclear structure in unstimulated HEK293 cells stably transfected with TLR4 and its coreceptors MD2 and CD14 (HEK293-MCT) cells ( Fig. 2c ). After 10 min LPS treatment, TMED7 can be seen in small endosomal-like structures. After 20 and 30 min LPS treatment, TMED7 can be seen in the limiting membrane of enlarging endosomal-like structures ( Fig. 2c , arrows). After 40 min LPS stimulation, TMED7 can be seen gathered in structures reminiscent of late endosomes. After 60 min LPS treatment, TMED7 can be seen in a reticular pattern reminiscent of TAG localization. 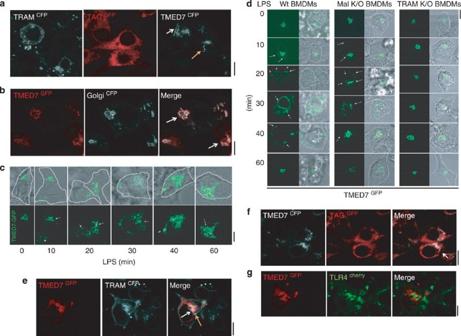Figure 2: TMED7 trafficks from the Golgi into maturing endosomes in response to LPS. Confocal images showing (a) TRAMCFP, TAGGFPand TMED7CFPare differentially localized within HEK293 cells. (b) TMED7GFP(represented in red) co-localising with GolgiCFPin HEK293 cells. (c) HEK293-MCT cells were transfected with TMED7GFP(represented in green) and stimulated with LPS (250 ng ml−1) over 10, 20, 30, 40 and 60 min. Cells were then fixed and visualized by confocal microscopy, original magnification ×60. (d) Wild-type (Wt, left-hand panel), Mal knockout (KO; middle panel) and TRAM KO (right-hand panel) iBMDMs were transfected with TMED7GFP(represented in green) and treated with LPS (250 ng ml−1) for 10, 20, 30, 40 and 60 min, respectively, fixed and visualized by confocal microscopy, original magnification ×60. Arrows indicate endosome-like structures. Confocal images showing localization of (e) TMED7GFPand TRAMCFP, (f) TMED7CFPand TAGGFP, and (g) TMED7GFPand TLR4cherryintracellularly in resting cells. (a,b,e–g) The CFP tag is represented in cyan and the GFP tag is represented in red, the cherry tag is represented in green. Confocal data is representative of at least three experiments. Scale bars indicate 10 μM. Figure 2: TMED7 trafficks from the Golgi into maturing endosomes in response to LPS. Confocal images showing ( a ) TRAM CFP , TAG GFP and TMED7 CFP are differentially localized within HEK293 cells. ( b ) TMED7 GFP (represented in red) co-localising with Golgi CFP in HEK293 cells. ( c ) HEK293-MCT cells were transfected with TMED7 GFP (represented in green) and stimulated with LPS (250 ng ml −1 ) over 10, 20, 30, 40 and 60 min. Cells were then fixed and visualized by confocal microscopy, original magnification ×60. ( d ) Wild-type (Wt, left-hand panel), Mal knockout (KO; middle panel) and TRAM KO (right-hand panel) iBMDMs were transfected with TMED7 GFP (represented in green) and treated with LPS (250 ng ml −1 ) for 10, 20, 30, 40 and 60 min, respectively, fixed and visualized by confocal microscopy, original magnification ×60. Arrows indicate endosome-like structures. Confocal images showing localization of ( e ) TMED7 GFP and TRAM CFP , ( f ) TMED7 CFP and TAG GFP , and ( g ) TMED7 GFP and TLR4 cherry intracellularly in resting cells. ( a , b , e – g ) The CFP tag is represented in cyan and the GFP tag is represented in red, the cherry tag is represented in green. Confocal data is representative of at least three experiments. Scale bars indicate 10 μM. Full size image We next investigated whether Mal or TRAM might have a role in the changing location of TMED7 after LPS stimulation. The location of TMED7 in wild-type immortalized bone marrow-derived macrophages (iBMDM) changes following LPS stimulation, in a similar manner to that observed in the HEK293-MCT cells ( Fig. 2d ). TMED7 moves from a Golgi-like perinuclear structure into the endosome-like structures following LPS stimulation, before appearing in a reticular perinuclear structure 60 min post-LPS treatment. This pattern of TMED7 movement was mirrored in Mal-deficient iBMDMs. In TRAM-deficient iBMDMs, TMED7 remained in a Golgi-like perinuclear location, despite LPS stimulation. This suggests that TRAM engagement is required to initiate the movement of TMED7 upon LPS stimulation. Consistent with these observations, TMED7 was found to co-localize with TRAM intracellularly ( Fig. 2e , white arrow), but not at the plasma membrane ( Fig. 2e , orange arrow). It was also shown to co-localize with TAG to a small extent basally ( Fig. 2f , arrow). TMED7 was not found co-localized with TLR4 in resting cells ( Fig. 2g ). Because of the high level of co-localization of TMED7 with TRAM, and the apparent movement of TMED7 after LPS treatment, we examined whether TMED7 had a role during LPS signalling in the EEA1-positive early endosome. In resting cells, TMED7 does not appear on the limiting membrane of early endosomes. Upon 15-min LPS treatment, although the extent of co-localization was minimal, TMED7 could be found in microdomains on enlarged early endosomes. After 30 min LPS treatment, TMED7 partially localized to the limiting membrane of EEA1-positive endosomes ( Fig. 3a ). We next examined the localization of TMED7, TRAM and TLR4 in HEK293 cells stably expressing TLR4-mCherry. Under basal conditions, TMED7 co-localizes with TRAM, but not with TLR4 ( Fig. 2e and g ). After 20 min LPS treatment, TLR4 and TRAM could be found close to TMED7 containing endosomes, and after 40 and 60 min LPS treatment, TRAM and TLR4 can be found clearly colocalizing with TMED7 ( Fig. 3b , arrows). To confirm the confocal microscopy data, we investigated if TRAM and TMED7 could interact. There is no suitable antibody towards endogenous TRAM, so we investigated if TRAM-GFP could interact with endogenous TMED7. Fig. 3c demonstrates that TMED7 and TRAM can interact (lane 2) and, interestingly, this interaction increases upon LPS stimulation (lane 3). To determine the specificity of this interaction, we utilized TMED1 and found that TMED1 could not interact with TRAM ( Fig. 3d , lane 5). 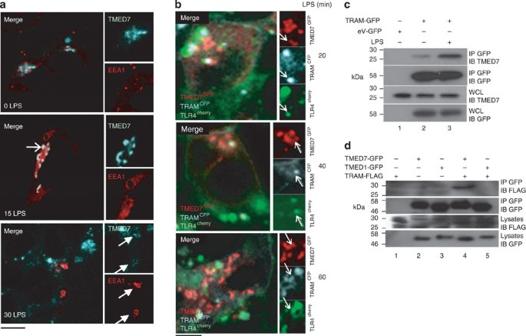Figure 3: TMED7 co-localizes with TRAM and TLR4 after LPS treatment. (a) HEK293 cells stably expressing TLR4 and transiently transfected with MD2, CD14, TMED7CFPand the early-endosome marker EEA1GFPwere first imaged untreated and then stimulated with LPS (250 ng ml−1) for 15 and 30 min as indicated. (b) HEK293 cells stably expressing TLR4cherryand transiently transfected with MD2, CD14, TRAMCFPand TMED7GFPwere stimulated with LPS (250 ng ml−1) for 20, 40 and 60 min. (a,b) TMED7GFPis represented in red; EEA1CFPand TRAMCFPare represented in cyan, and TLR4cherryis represented in green. Confocal data is representative of three experiments, a minimum of 50 cells were analysed. (c,d) Immunoprecipitation and immunoblot analysis of HEK293 cells transfected with (c) TRAM-GFP or eV-GFP, followed by LPS (100 ng ml−1) stimulation for 30 min or (d) TMED7-GFP, or TMED1-GFP and TRAM-FLAG. Scale bars indicate 10 μM. Figure 3: TMED7 co-localizes with TRAM and TLR4 after LPS treatment. ( a ) HEK293 cells stably expressing TLR4 and transiently transfected with MD2, CD14, TMED7 CFP and the early-endosome marker EEA1 GFP were first imaged untreated and then stimulated with LPS (250 ng ml −1 ) for 15 and 30 min as indicated. ( b ) HEK293 cells stably expressing TLR4 cherry and transiently transfected with MD2, CD14, TRAM CFP and TMED7 GFP were stimulated with LPS (250 ng ml −1 ) for 20, 40 and 60 min. ( a , b ) TMED7 GFP is represented in red; EEA1 CFP and TRAM CFP are represented in cyan, and TLR4 cherry is represented in green. Confocal data is representative of three experiments, a minimum of 50 cells were analysed. ( c , d ) Immunoprecipitation and immunoblot analysis of HEK293 cells transfected with ( c ) TRAM-GFP or eV-GFP, followed by LPS (100 ng ml −1 ) stimulation for 30 min or ( d ) TMED7-GFP, or TMED1-GFP and TRAM-FLAG. Scale bars indicate 10 μM. Full size image TMED7 inhibits the MyD88-independent TLR4 pathway TMED7 co-localizes with TRAM and TAG basally, and with TLR4 after LPS treatment. We next examined a role for TMED7 in TLR4 signalling. TMED7 overexpression in HEK293-MCT cells could not induce an interferon-sensitive response element (ISRE)- or κB-linked reporter gene ( Fig. 4a and b, respectively). LPS stimulation activated the ISRE reporter gene, and this was inhibited by TMED7 overexpression ( Fig. 4a ). TMED7 overexpression had no effect on κB reporter gene activation by LPS ( Fig. 4b ). TMED7 overexpression did not affect the activation of ISRE in HEK293-TLR3 cells stimulated with PolyI:C ( Fig. 4c ), suggesting that TMED7 specifically inhibits the MyD88-independent TLR4 pathway. Overexpression of TRAM activated the ISRE reporter gene, but TMED7 co-expression prevented TRAM-induced ISRE activation ( Fig. 4d ). IRF3 phosphorylation occurred 60 min post-LPS stimulation, but TMED7 overexpression prevented this phosphorylation ( Fig. 4e ). TMED7 overexpression also reduces type 1 IFN levels following LPS stimulation ( Fig. 4f ). 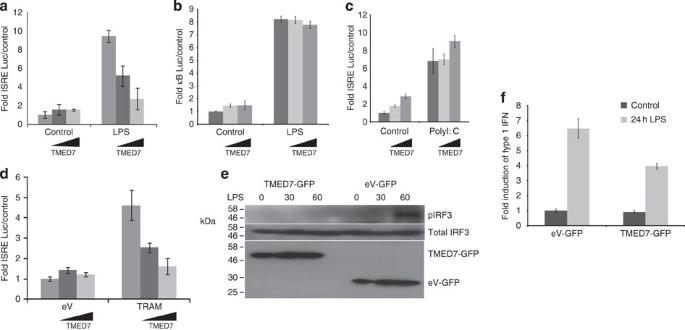Figure 4: TMED7 overexpression inhibits the TLR4 MyD88-independent signalling pathway. Luciferase activity was measured in HEK293 cells stably expressing TLR4, MD2 and CD14 (HEK293-MCT) (a,b), HEK293 cells stably expressing TLR3 (c) or HEK93 cells (d), transfected with the ISRE- (a,c,d) or κB-luciferase (b) reporter gene, the control renilla luciferase gene plus empty vector, or increasing amounts of plasmid expressing TMED7-GFP (10 and 50 ng). The cells were also transfected with TRAM-FLAG (d) or stimulated with or without (a,b) LPS (100 ng ml−1) or (c) poly(I:C) (25 μg ml−1) for 6 h. (e) HEK293-MCT cells transfected with eV-GFP or TMED7-GFP were stimulated with LPS (100 ng ml−1) for 0, 30 or 60 min. Cells were lysed and immunoblotted for total IRF3 or phospho-Ser-396 IRF3 (pIRF3). (f) Supernatants from HEK293-MCT cells transfected with ev–GFP or TMED7–GFP and stimulated with LPS (100 ng ml−1) for 24 h were incubated with HEK-blue IFN cells for 24 h. Levels of IFN present are represented as fold over unstimulated eV control. Data are representative of three separate experiments anda,b,c,dandfare presented as mean ± s.d. Figure 4: TMED7 overexpression inhibits the TLR4 MyD88-independent signalling pathway. Luciferase activity was measured in HEK293 cells stably expressing TLR4, MD2 and CD14 (HEK293-MCT) ( a , b ), HEK293 cells stably expressing TLR3 ( c ) or HEK93 cells ( d ), transfected with the ISRE- ( a , c , d ) or κB-luciferase ( b ) reporter gene, the control renilla luciferase gene plus empty vector, or increasing amounts of plasmid expressing TMED7-GFP (10 and 50 ng). The cells were also transfected with TRAM-FLAG ( d ) or stimulated with or without ( a , b ) LPS (100 ng ml −1 ) or ( c ) poly(I:C) (25 μg ml −1 ) for 6 h. ( e ) HEK293-MCT cells transfected with eV-GFP or TMED7-GFP were stimulated with LPS (100 ng ml −1 ) for 0, 30 or 60 min. Cells were lysed and immunoblotted for total IRF3 or phospho-Ser-396 IRF3 ( pIRF3 ). ( f ) Supernatants from HEK293-MCT cells transfected with ev–GFP or TMED7–GFP and stimulated with LPS (100 ng ml −1 ) for 24 h were incubated with HEK-blue IFN cells for 24 h. Levels of IFN present are represented as fold over unstimulated eV control. Data are representative of three separate experiments and a , b , c , d and f are presented as mean ± s.d. Full size image TMED7 knockdown potentiates the TRIF-dependent TLR4 pathway An small interfering RNA (siRNA) oligomer targeting the unique C terminus region of TMED7 was used, along with previously verified TRAM siRNA and TAG siRNA [9] . The specificity of the oligomers was confirmed in peripheral blood mononuclear cells (PBMCs) and THP1 cells ( Fig. 5a and b ). TRAM knockdown inhibited the ability of LPS to activate the κB and ISRE reporter genes ( Fig. 5c ). Similar to TAG, TMED7 knockdown enhanced the ability of LPS to induce the ISRE reporter gene, but had no effect on the κB reporter gene, again suggesting that TMED7 inhibits the MyD88-independent pathway. TRAM overexpression activated the ISRE reporter gene, and TAG or TMED7 knockdown potentiated TRAM's ability to activate this gene ( Fig. 5d ). 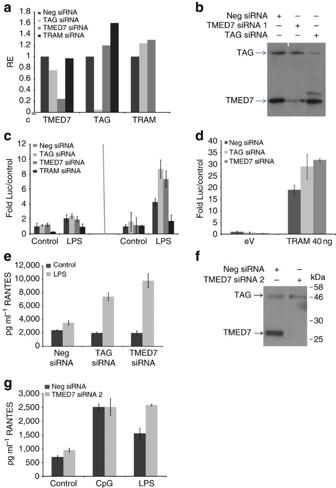Figure 5: Knockdown of TMED7 potentiates the TLR4 MyD88-independent signalling pathway. (a) TRAM, TAG and TRAM were knocked down in hPBMCs using siRNA and quantitative reverse transcription–PCR was performed to determine knockdown of TRAM, TAG and TRAM. (b) Whole-cell lysates from THP1 cells, transfected with control siRNA, TMED7 siRNA or TAG siRNA, were isolated and analysed by western blot using TICAM2 antibody. (c,d) Luciferase reporter assay for the activity of κB-luciferase (c, left-hand panel) or ISRE-luciferase (c, right-hand panel, andd) were performed in HEK293-MCT cells transfected with 20 nM control siRNA, TRAM siRNA, TAG siRNA or TMED7 siRNA. The cells were either (c) left untreated, stimulated with LPS (100 ng ml−1) for 24 h or (d) transfected with TRAM-FLAG. Results are normalized to renilla luciferase activity and are presented relative to unstimulated cells containing empty vector. (e) Whole-cell lysates from THP1 cells, transfected with control siRNA or TMED7 siRNA 2, were isolated and analysed by western blot using TICAM2 antibody. (f) 20 nM control siRNA, TAG siRNA or TMED7 siRNA were transfected into human PMBCs. After 48 h transfection, the cells were left untreated or treated with LPS (50 ng ml−1) for 24 h. An enzyme-linked immunosorbent assay of CCL5 (RANTES) was performed. (g) Control siRNA (20 nM), TMED7 siRNA 2 were transfected into human PMBCs. After 48 h transfection, the cells were left untreated or treated with LPS (50 ng ml−1) or CpG (5 μg ml−1) for 24 h. An enzyme-linked immunosorbent assay of CCL5 (RANTES) was performed. Data are representative of three separate experiments andc,d,eandgare presented as mean ± s.d. Figure 5: Knockdown of TMED7 potentiates the TLR4 MyD88-independent signalling pathway. ( a ) TRAM, TAG and TRAM were knocked down in hPBMCs using siRNA and quantitative reverse transcription–PCR was performed to determine knockdown of TRAM, TAG and TRAM. ( b ) Whole-cell lysates from THP1 cells, transfected with control siRNA, TMED7 siRNA or TAG siRNA, were isolated and analysed by western blot using TICAM2 antibody. ( c , d ) Luciferase reporter assay for the activity of κB-luciferase ( c , left-hand panel) or ISRE-luciferase ( c , right-hand panel, and d ) were performed in HEK293-MCT cells transfected with 20 nM control siRNA, TRAM siRNA, TAG siRNA or TMED7 siRNA. The cells were either ( c ) left untreated, stimulated with LPS (100 ng ml −1 ) for 24 h or ( d ) transfected with TRAM-FLAG. Results are normalized to renilla luciferase activity and are presented relative to unstimulated cells containing empty vector. ( e ) Whole-cell lysates from THP1 cells, transfected with control siRNA or TMED7 siRNA 2, were isolated and analysed by western blot using TICAM2 antibody. ( f ) 20 nM control siRNA, TAG siRNA or TMED7 siRNA were transfected into human PMBCs. After 48 h transfection, the cells were left untreated or treated with LPS (50 ng ml −1 ) for 24 h. An enzyme-linked immunosorbent assay of CCL5 (RANTES) was performed. ( g ) Control siRNA (20 nM), TMED7 siRNA 2 were transfected into human PMBCs. After 48 h transfection, the cells were left untreated or treated with LPS (50 ng ml −1 ) or CpG (5 μg ml −1 ) for 24 h. An enzyme-linked immunosorbent assay of CCL5 (RANTES) was performed. Data are representative of three separate experiments and c , d , e and g are presented as mean ± s.d. Full size image The effect of TMED7 knockdown on CCL5 (RANTES) production, an ISRE-dependent gene, following LPS treatment was examined in human PBMCS (hPBMCs). Knocking down TMED7, like TAG, increased RANTES production in response to LPS ( Fig. 5e ). A second siRNA towards TMED7 also reduced TMED7 protein levels ( Fig. 5f ) and enhanced the levels of RANTES produced in response to LPS ( Fig. 5g ), ensuring the enhancement was not due to off-target effects. TMED7's inhibitory role appears to be specific for TLR4 as the levels of RANTES production following stimulation with the TLR9 ligand, CpG were unaffected by TMED7 knockdown ( Fig. 5g ). TMED7 trafficks away from Rab11a positive membranes Husebye et al . [11] have demonstrated that Rab11a is essential for the movement of TLR4 to the ERC and recruitment of both TLR4 and TRAM to the E. coli -containing phagosomes for the activation of the IRF3 pathway upon E. coli or LPS treatment, with little effect on the NF-κB pathway. The specificity of Rab11a for the IRF3 pathway led us to investigate possible interplay between Rab11a and TMED7. TMED7-GFP and Rab11a-CFP were co-expressed in HEK293 cells. In resting cells, TMED7 could be found localized to microdomains on Rab11a-positive endosomal structures ( Fig. 6a ). Following 20 min of LPS treatment, the co-localization of TMED7 and Rab11a appeared to increase, with clear endosomal structures double-positive for both Rab11a and TMED7. Following 40 min of LPS stimulation, co-localization between TMED7 and Rab11a decreased because of TMED7's emerging reticular pattern. We examined whether TAG-GFP could co localize with Rab11a. In resting cells, TAG co localized with Rab11a, but not to the same extent as TMED7 ( Fig. 6b ), and co-localization was minimal after 40 min LPS treatment. To determine if Rab11a has a direct role in the localization of TMED7 in the cell, we knocked down Rab11a using siRNA. In control cells, TMED7 appears in its Golgi-like pattern early into LPS treatment, moving to a more endosomal pattern before appearing more reticular in pattern, following 30 to 60 min LPS treatment ( Fig. 6c ). In cells where Rab11a is knocked down, TMED7 appears to remain in the Golgi even after LPS treatment ( Fig. 6c ). Following 60 min LPS treatment, TMED7 no longer co localizes with a trans-Golgi-network (TGN) marker in control cells. Conversely, in cells where Rab11a has been knocked down, TMED7 still co-localizes with the TGN marker ( Fig. 6d ). This suggests that Rab11a is not required for the retention of TMED7 in the TGN, but is required for the trafficking of TMED7 away from the Golgi after LPS stimulation. 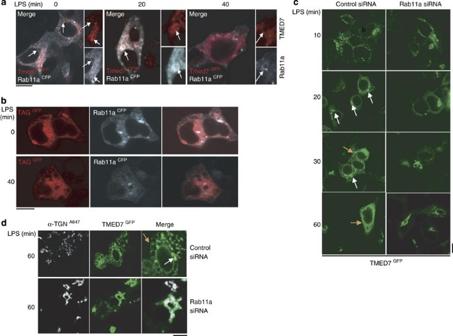Figure 6: Rab11a is required for the trafficking of TMED7 in response to LPS. (a,b) Live cell confocal images of HEK293 cells stably expressing TLR4 and transiently transfected with MD2, CD14, the ERC marker Rab11aCFPand (a) TMED7GFPor (b) TAGGFPwere first imaged untreated and then stimulated with LPSCy5(250 ng ml−1) for (a) 20 and 40 min or (b) 40 min. TMED7GFPand TAGGFPare represented in red, Rab11aCFPis represented in white. (c,d) HEK293 cells stably expressing TLR4 and transiently transfected with MD2, CD14 and TMED7GFPwere transfected with either control siRNA or siRNA targeting Rab11a, and then stimulated with LPS for the times indicated. (d) Cells were fixed and stained with an antibody to the TGN, and further incubated with a secondary antibody conjugated to Alexafluor-647. (c,d) TMED7GFPis represented in green, TGN647in white. Data are representative of three independent experiments, with a minimum of 30 cells analysed. Scale bars indicate 10 μM. Figure 6: Rab11a is required for the trafficking of TMED7 in response to LPS. ( a , b ) Live cell confocal images of HEK293 cells stably expressing TLR4 and transiently transfected with MD2, CD14, the ERC marker Rab11a CFP and ( a ) TMED7 GFP or ( b ) TAG GFP were first imaged untreated and then stimulated with LPS Cy5 (250 ng ml −1 ) for ( a ) 20 and 40 min or ( b ) 40 min. TMED7 GFP and TAG GFP are represented in red, Rab11a CFP is represented in white. ( c , d ) HEK293 cells stably expressing TLR4 and transiently transfected with MD2, CD14 and TMED7 GFP were transfected with either control siRNA or siRNA targeting Rab11a, and then stimulated with LPS for the times indicated. ( d ) Cells were fixed and stained with an antibody to the TGN, and further incubated with a secondary antibody conjugated to Alexafluor-647. ( c , d ) TMED7 GFP is represented in green, TGN 647 in white. Data are representative of three independent experiments, with a minimum of 30 cells analysed. Scale bars indicate 10 μM. Full size image TMED7 trafficks to the late endosome where it encounters TAG As mentioned above, to limit TLR4 signalling after the initial LPS stimulation, TRAM and TLR4 are known to move to Rab7-positive late endosomes, where the complex encounters TAG. TAG then disrupts the TRIF–TRAM interaction and promotes TLR4 degradation, resulting in the inhibition of the IRF3 pathway [9] . We investigated whether TMED7 could be found in Rab7-positive late endosomes. TMED7 co-localizes to a minor extent with Rab7a in resting cells ( Fig. 7a ). After 60 min LPS stimulation, co-localization of TMED7 and Rab7a increased substantially, with large TMED7 domains found on the limiting membrane of Rab7a-positive endosomes that also contained TLR4, both in the membrane and the lumen ( Fig. 7a , arrows). 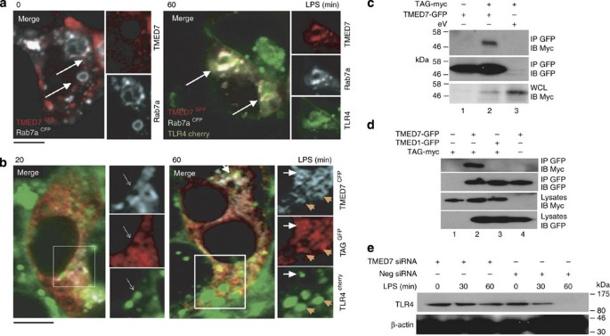Figure 7: TMED7 trafficks to the late endosome where it encounters TAG. (a,b) HEK293 cells stably expressing TLR4cherryand transiently expressing MD2, CD14, TMED7GFPand Rab7aCFPwere imaged untreated (a, left-hand panel) and then stimulated with LPSCy5(250 ng ml−1) for 60 min (a, right-hand panel), TMED7GFPis represented in red, Rab7aCFPin cyan and TLR4cherryin green. A total of 46 cells were analysed over time. (b) HEK293 cells stably expressing TLR4cherryand transiently expressing MD2, CD14, TMED7CFPand TAGGFPwere stimulated with LPS (250 ng ml−1) for 20 (b, left-hand panel) or 60 min (b, right-hand panel). TMED7CFPis represented in cyan, TAGGFPin red and TLR4cherryin green. A total of 44 cells were analysed. Scale bars indicate 10 μM. (c,d) Immunoprecipitation and immunoblot analysis of HEK293 cells transfected with (c) TMED7-GFP or ev-GFP and TAG-myc, or (d) TMED7-GFP or TMED1-GFP and TAG-myc. (e) THP-1 cells transfected with 20 nM TMED7 siRNA or a negative scrambled siRNA. After 48 h transfection, cells were stimulated with LPS (100 ng ml−1). Lysates were immunoblotted for TLR4 or β-actin. (c–e) The immunoprecipitating antibodies (IP) and the immunoblotting antibodies (IB) are listed beside the appropriate blot. Data are representative of three independent experiments. Figure 7: TMED7 trafficks to the late endosome where it encounters TAG. ( a , b ) HEK293 cells stably expressing TLR4 cherry and transiently expressing MD2, CD14, TMED7 GFP and Rab7a CFP were imaged untreated ( a , left-hand panel) and then stimulated with LPS Cy5 (250 ng ml −1 ) for 60 min ( a , right-hand panel), TMED7 GFP is represented in red, Rab7a CFP in cyan and TLR4 cherry in green. A total of 46 cells were analysed over time. ( b ) HEK293 cells stably expressing TLR4 cherry and transiently expressing MD2, CD14, TMED7 CFP and TAG GFP were stimulated with LPS (250 ng ml −1 ) for 20 ( b , left-hand panel) or 60 min ( b , right-hand panel). TMED7 CFP is represented in cyan, TAG GFP in red and TLR4 cherry in green. A total of 44 cells were analysed. Scale bars indicate 10 μM. ( c , d ) Immunoprecipitation and immunoblot analysis of HEK293 cells transfected with ( c ) TMED7-GFP or ev-GFP and TAG-myc, or ( d ) TMED7-GFP or TMED1-GFP and TAG-myc. ( e ) THP-1 cells transfected with 20 nM TMED7 siRNA or a negative scrambled siRNA. After 48 h transfection, cells were stimulated with LPS (100 ng ml −1 ). Lysates were immunoblotted for TLR4 or β-actin. ( c – e ) The immunoprecipitating antibodies (IP) and the immunoblotting antibodies (IB) are listed beside the appropriate blot. Data are representative of three independent experiments. Full size image Considering TAG is also found in Rab7a-positive late endosomes, where it encounters TLR4 after LPS stimulation, we examined whether TMED7 could co-localize with TAG and TLR4. We had seen TMED7 co-localize with TAG to some extent, but not with TLR4 in resting cells ( Fig. 2f and g ). After 20 LPS stimulation, TMED7 appeared more reticular in its expression pattern and could be seen to co-localize with TAG and TLR4 ( Fig. 7b ). TMED7 and TLR4 could also be seen to co-localize in microdomains on TAG-positive endosomes, rather than coating the entire limiting membrane. Following 60 min LPS stimulation, in addition to endosomes where TMED7/TLR4/TAG were present on the limiting membrane ( Fig. 7b , white arrows), TLR4 could also be visualized in the lumen of TAG- and TMED7-positive late endosomal structures ( Fig. 7b , orange arrows). We performed an immunoprecipitation assay to confirm that TMED7 and TAG interact ( Fig. 7c , lane 2). TMED1, another member of the TMED family, could not interact with TAG, confirming the specificity of the TMED7–TAG interaction ( Fig. 7d ). TAG is essential for the degradation of TLR4 in late endosomes [9] . We investigated if TMED7 was also vital for TLR4 degradation following LPS stimulation. After 60 min LPS stimulation, THP1 cells transfected with a scrambled siRNA showed significant TLR4 degradation, whereas cells transfected with TMED7 siRNA showed little or no TLR4 degradation ( Fig. 7e ). This demonstrates that TMED7 is also required for TLR4 degradation following LPS stimulation. TMED7 facilitates the displacement of TRAM from TRIF by TAG We investigated if TMED7 could disrupt the interaction between TRIF and TRAM in a similar manner to TAG. Haemagglutinin-tagged TRIF and TRAM-FLAG were overexpressed in HEK293 cells with or without TMED7-GFP or TAG-myc. TMED7 overexpression resulted in a reduction in the interaction between TRIF and TRAM ( Fig. 8a ), although not as efficiently as TAG ( Fig. 8a ). To determine if TAG and TMED7 work in cooperation, we examined if TAG could still disrupt the TRIF/TRAM pathway in the absence of TMED7. When TMED7 was knocked down using siRNA, TAG could no longer disrupt the TRIF–TRAM complex ( Fig. 8b ), suggesting that TMED7 is indeed required for the inhibition of the MyD88-independent pathway by TAG. 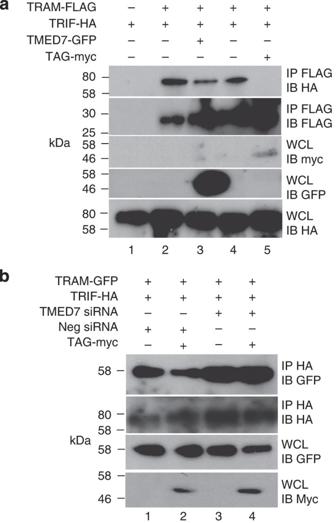Figure 8: TMED7 enables the disruption of the TRAM–TRIF complex. (a) HEK293 cells transfected with TRAM-FLAG and TRIF-(haemagglutinin) HA in the presence or absence of TMED7-GFP or TAG-myc. (b) HEK293 cells were transfected with TMED7 siRNA, and TRAM-FLAG and TRIF-HA in the presence or absence of TAG-myc. The immunoprecipitating antibodies (IP) and the immunoblotting antibodies (IB) are listed beside the appropriate blot. Data are representative of three independent experiments. Figure 8: TMED7 enables the disruption of the TRAM–TRIF complex. ( a ) HEK293 cells transfected with TRAM-FLAG and TRIF-(haemagglutinin) HA in the presence or absence of TMED7-GFP or TAG-myc. ( b ) HEK293 cells were transfected with TMED7 siRNA, and TRAM-FLAG and TRIF-HA in the presence or absence of TAG-myc. The immunoprecipitating antibodies (IP) and the immunoblotting antibodies (IB) are listed beside the appropriate blot. Data are representative of three independent experiments. Full size image This study identifies for the first time a role for TMED7 in the negative regulation of TLR4 signalling by demonstrating that TMED7 facilitates the inhibition of the MyD88-independent pathway by TAG. TAG possesses the GOLD domain of TMED7 and the TIR domain of TRAM, because of the read-through from the tmed7 gene into the ticam2 gene. GOLD domain containing proteins are known to be involved in vesicular transport, but several recent papers have suggested novel roles for these proteins. Of particular interest is emerging evidence of the role TMED family members might have in innate immune regulation. A homologue of TMED in Drosophila , termed logjam, has been implicated in negatively regulating a large number of immune-related genes, including many targets of the Toll and Imd signalling pathways [20] . In addition, TMED1 has been shown to interact with the IL-1R/TLR member ST2 [21] . Although a function has yet to be assigned to this interaction, it is particularly interesting, as ST2 negatively regulates TLR4 [22] . Our findings with TMED7 are the first to characterize a role for a TMED family member in the mammalian immune system and further emphasize the likely importance of TMED members in immunoregulation. Confocal microscopy revealed TMED7 displays a distinct subcellular localization to both TRAM and TAG. TMED7 localizes mainly to the Golgi in resting cells, whereas TAG displays a more reticular pattern localizing to the ER. TRAM is found in the plasma membrane and intracellularly in small endosomes. The bipartite motif at the N terminus of TRAM is essential for its localization [23] but TAG and TMED7 do not possess this motif. It was previously thought that, because of a predicted transmembrane domain at the C terminus of TMED7, the GOLD domain of TMED7 would project into the lumen of the Golgi, leaving a short N-terminal tail protruding into the cytosol [24] . However, our investigations suggest that both TMED7 and TAG have a predicted transmembrane-spanning region in their N termini, and studies revealed that it is this predicted N-terminus transmembrane domain that is responsible for TMED7's ability to span the membrane, and that the GOLD domain and C terminus of TMED7 project into the cytosol. This would allow for a homotypic interaction between the GOLD domains of TMED7 and TAG in the cytosol and provides a possible explanation for why TAG contains TMED7 within its sequence. The regulation of the location of the components of the TLR4 signalling pathway is emerging as a key feature of TLR4 function and Rab family members have been implicated in this process. TLR4 signals through the MyD88-dependent pathway at the plasma membrane. Rab10 has been shown to act as a positive regulator of TLR4 signalling by promoting transport of TLR4 from the Golgi to the plasma membrane [6] . Once engaged by LPS, TLR4 moves into early endosomes where it signals through the MyD88-independent pathway. Rab7b has been shown to act as a negative regulator by promoting the movement of TLR4 to late endosomes, where TLR4 is degraded [8] . Husebye et al . [11] have shown that Rab11a is essential for the trafficking of TLR4, along with TRAM and IRF3, from the Rab11a-positive ERC to E. coli - containing phagosomes. Suppression of Rab11a reduces TLR4 levels in the ERC and on the phagosomes, resulting in a reduction in IRF3 signalling in response to LPS or E. coli . This suggests that TLR4 can signal from Rab11a-positive endosomes, as well as EEA1-positive early endosomes. TMED7 is not present at the plasma membrane where TLR4 signals through the MyD88-dependent pathway. It is also absent in early endosomes, where TLR4 signals via TRAM and TRIF, until 30 min after LPS stimulation. TMED7 co-localizes extremely well with intracellular TRAM, even in resting cells; however, TLR4 is not found with TMED7 in resting cells, indicating that TRAM localizes to different pools intracellularly, one pool in the early endosomes containing TLR4 and another pool, probably Rab11a positive, containing TMED7. Following LPS stimulation, TMED7 rapidly trafficks away from the Golgi towards the maturing endosomal network, eventually residing in a reticular pattern throughout the cell. This movement of TMED7 occurs in both a TRAM- and Rab11a-dependent manner, indicating that TMED7 responds to LPS stimulation through the MyD88-independent pathway, and requires Rab11a for its initial removal from the Golgi. This correlates well with the increased appearance of TMED7 in Rab11a-positive endosomes early, and disappearance of TMED7 from Rab11a-positive endosomes later, after LPS treatment. Furthermore, TMED7 is absent in EEA1-positive early endosomes until 30 min after LPS treatment, approximately the same time we begin to see the appearance of small amounts of co-localization of TMED7 with both TRAM and TLR4. Later on after LPS treatment, TMED7 can be found to localize to Rab7a-positive late endosomes with similar kinetics to the co-localization of both TRAM and TAG with TMED7 in late endosomes, suggesting that TMED7, TAG and TRAM all co-localize at the Rab7a-positive late endosome, where TLR4 can be found both in the limiting membrane and in the lumen of the endosomes. The mechanism of interaction between TMED7 and TRAM will need to be investigated further, and may require TAG as an intermediate, which might explain why the interaction between TRAM and TMED7 increases upon LPS stimulation. TAG overexpression disrupts the interaction between TRIF and TRAM. TMED7 appears to facilitate this disruption of the TRAM–TRIF complex by TAG. The lack of TMED7 and TAG in early endosomes would allow the TRIF-TRAM pathway to signal after the initial TLR4 ligation. TMED7 may facilitate the movement of TLR4/TRAM to Rab7-positive endosomes, where TMED7 and TAG work in partnership to inhibit the pathway by disrupting the TRIF–TRAM interaction and promoting TLR4 degradation. There is very limited literature on TMED7. Jerome et al . [13] demonstrated that TMED2 is found in a complex with TMED10 and TMED7, and that the presence of TMED2 is essential for their stability [25] . Therefore, the knockdown of TMED7 using siRNA is likely to affect the stability of other TMED family members. The role of these other TMED family members in TLR signalling will need to be investigated. TMED7 has also been shown to be upregulated in a metastatic nasopharyngeal carcinoma cell line, which could be immunosuppressive [26] . A role for TMED7 in modulating TLR4 in anti-tumour immunity could therefore be worth exploring. In conclusion, our study identifies a role for TMED7 as a specific inhibitor of the MyD88-independent TLR4 signalling pathway, by facilitating the disruption of the TRIF/TRAM complex by TAG. Further analysis of the role of the TMED family in the regulation of the IL1R/TLR family is likely to provide new insights in to the control of innate immunity. Therapeutic implications of these data could be in improved vaccine adjuvancy, as targeting TMED7 along with TAG may allow for specific immunopotentiation of TLR4 induction of IFN-sensitive genes without aggravating the more inflammatory arm of the TLR4 gene induction. Reagents The TLR agonists used were poly(I:C) (Amersham Biosciences) and LPS (TLRGrade™, Alexis). Cy5-labelling of LPS was performed as previously described [10] . SiRNA oligonucleotides (Qiagen) used were: negative scrambled oligonucleotide: 5′-AATATAATTCAATCACACAAC-3′, siRNA targeting N terminal of Tram: 5′-AAACCCATTATAAATATCCAA-3′, siRNA targeting N terminal of TAG: 5′-AACCGTTTAAGAGAAGCTCAA-3′, siRNA targeting C terminal of TMED7: 5′-AACCACCACAACTCGTGTTGG-3′, siRNA2 targeting C terminal of TMED7: 5′-GCCCTCATTCTTCTGGTGG-3′ and Hs_RAB11A_5 HP validated siRNA (QIAGEN). TRAM-CFP, TRAM-FLAG were obtained from K. Fitzgerald, University of Massachusetts, Boston, USA; Rab7a-CFP was obtained from M. Zerial, Dresden, Germany. Golgi-CFP, EEA1-CFP were obtained from Harald Stanmark, The Norwegian Radium Hospital, Oslo, Norway. EEA1-GFP, ER-CFP (targeting the sequence of calreticulin fused to CFP) were purchased from Clontech, CA, USA. Haemagglutinin-tagged TRIF was obtained from C. Basler, Mount Sinai School of Medicine, New York. TMED7-GFP, TMED7-CFP were purchased from GeneCopoeia, Rockville, USA. pIRF3 (Ser396) antibody was purchased from Cell Signaling and the total IRF3 antibody (FL-425) was purchased from Santa Cruz. Endogenous TMED7 and TAG were examined using the TICAM2 antibody (Sigma HPA008960). This antibody detects the GOLD domain of TMED7 and TAG, but does not detect TRAM. The specificity of this antibody was tested using siRNA towards TMED7 and TAG, confirming that the two bands detected are in fact TMED7 and TAG ( Supplementary Fig S2 ). Antibodies were used at a final concentration of 0.2 μg ml −1 . Reverse transcription–PCR Total RNA from cells seeded in 12- or 6-well plates was extracted with the RNAeasy kit (Qiagen) and was reverse-transcribed by SuperScript II Reverse Transcriptase (Invitrogen) according to the manufacturer's protocol. This cDNA or the cDNA from the human adult normal tissue cDNA panel (Biochain) served as template for amplification of target genes, along with the 'housekeeping' gene GAPDH , by real-time PCR with Platinum SYBR Green qPCR SuperMix-UDG (Invitrogen) to determine the relative amounts of TMED7, Tram and TAG mRNA. The ABI 7900HT system (Applied Biosystems) was used for real-time PCR, and the cycling threshold method (2 −(ΔΔCt) ) was used for relative quantification by comparative method after normalization to GAPDH expression. The primers used were: TAG forward 5′-TGGAATCTGCCTGTGTTTCA-3′; reverse 5′-TGTTGGCCCCTCTGTTGTAT-3′; TRAM forward 5′-TTCCTGCCCTCTTTCTCTCTC-3′; reverse 5′-AACATCTCTTCCACGCTCTGA-3′ and TMED7 forward 5′-TTGGAGAAGACCCACCTTTG-3′, reverse 5′-GCCCTATGCTAACCACCAGA-3′. Confocal imaging HEK293 cell lines that stably expressed human TLR4 cherry were used and cultured in Dulbecco's modified Eagle's medium supplemented with 10% fetal calf serum and 0.5 mg ml −1 G418 and transfected using GeneJuice (Novagene) according to the manufacturer's protocol. iBMDM cells were cultured as above and transfected using lipofectamine (Invitrogen) according to the manufacturer's protocol. LPS was sonicated for 5 min and preincubated in serum-containing medium at 37 °C for 5 min before being added to cells. For confocal imaging, the cells were seeded on 35-mm glass bottom γ-irradiated tissue cell dishes (MatTek Corporation) and buffered with 25 mM HEPES (4-(2-hydroxyethyl)-1-piperazineethanesulfonic acid) buffer just before stimulation. LPS CY5 (250 ng ml −1 ) was used. Formaldehyde (2%) was used to fix cells if required. Images of live cells were captured at 37 °C, using an Axiovert 100-M microscope equipped with a Zeiss LSM 510 META scanning unit and a 1.4 NA ×63 plan apochromat objective. Dual or triple colour images were acquired one active laser line at a time to avoid cross-bleeding between channels. Coimmunoprecipitation and immunoblot analysis HEK293 cells or HEK293 cells stably transfected with MD2, CD14 and TLR4 (HEK293-MCT) (2.5×10 6 cells per 10-cm dish) were transfected with the indicated plasmids, where the total amount of DNA (8 μg) was kept constant using relevant empty vector. Wherever TRAM and TAG or TMED7 were co-expressed, two transfections were performed, with TRAM being expressed 24 h before the introduction of TAG or TMED7. This was done to ensure optimal expression of both proteins. After 24 or 48 h, cells were lysed as per the manufacturer's protocol. Flag ® M2 agarose beads (Sigma) or GFP-Trap beads (Chromotek) were incubated with cell lysates for 2 h at 4 °C. After the beads were washed, the immune complexes were eluted using 50 μl 5×Laemalli sample buffer, separated by SDS–polyacrylamide gel electrophoresis (PAGE), and proteins were detected by western blotting using relevant antibody: GFP-B2 (SC-9996) or c-Myc (9E10) from Santa Cruz Biotechnologies, FlagM2 (Sigma F3165), or HA (Covance MMS-101R)). Antibodies were used at a final concentration of 0.2 μg ml −1 . Reporter gene assays HEK293, HEK-TLR3 and HEK293-MCT cells (1×10 5 cells per ml) were seeded into 96-well plates and transfected 24 h later with expression vectors and luciferase reporter genes using GeneJuice (Novagen). Reporter genes used were for NF-κB and ISRE. In all cases, 40 ng per well of phRL-TK reporter plasmid (Promega) was cotransfected to allow normalization of data for transfection efficiency. The total amount of DNA per transfection was kept constant at 220 ng by the addition of pcDNA3.1 (Stratagene). After 18 h, cells were treated with TLR ligand, and 6 h later, reporter gene activity was measured. All reporter assays were done in triplicate and data were expressed as 'relative stimulation' (mean±s.d.) over the non-stimulated empty vector control, for a representative experiment, a total of three separate experiments being carried out. Measurement of type 1 IFN HEK293-MCT cells (1×10 5 cells per ml) were seeded into 96-well plates and were transfected 24 h later with TMED7 or eV. After 24 h, the cells were stimulated for 24 h with LPS. Supernatants (50 μl) were then removed and placed on HEK-blue IFN-α/β cells (Invivogen), which were seeded at 1×10 5 cells per ml in a 96-well plate 24 h previously. After 24 h, 20 μl supernatant was removed and added to 180 μl QUANTI-blue substrate and left at 37 °C for 30 min. The absorbance was measured at 625 nm. Transfection of HEK293 with siRNA HEK293-MCT cells (7.5×10 5 cells per 6-well plate) were transfected with indicated concentrations of siRNA oligonucleotides (Qiagen) using 4 μl Lipofectamine RNAiMax as per the manufacturer's instructions. After 24 h transfection, a second transfection was carried out using relevant reporter assay constructs. DNA (0.8 μg) was transfected per well, using Genejuice (Novagen). ISRE/κB-luciferase activity was measured 24 h later (described above). Transfection of hPBMC and measurement of hRANTES by ELISA The hPBMC were isolated from human blood and maintained in RPMI supplemented with 10% fetal calf serum, 2 mM L -glutamine, 1% penicillin/streptomycin solution (v/v). Cells (5×10 6 ) in 100 μl Buffer V (Amaxa Cell Line Nucleofector Kit V) were transfected with indicated amounts of siRNA (Qiagen) using Amaxa electroporation (Program Y-001, Version S3.4). Each sample was split into two wells containing prewarmed RPMI medium. After 24 h transfection, the medium was changed to reduce background cytokine levels and cells were stimulated with LPS for 24 h. Supernatants were collected and RANTES were determined by ELISA (R&D Systems, according to manufacturers recommendations). The use of these human samples complied with the regulations of Trinity College Dublin. Isolation of human CD14 + human monocytes PBMCs were isolated as above and then 300×10 6 cells were incubated with 300 μl CD14 microbeads (Mitlenyi Biotec) as per the manufacturer's instructions. The CD14 + monocytes were then separated out using a LS MACS column (Mitlenyi Biotec) and maintained in the same manner as the PBMCs above. Site-directed mutagenesis of TMED7 The QuikChange site-directed mutagenesis kit (Stratagene) was used to delete certain bases in the TMED7 gene. The manufacturer's instructions were followed. Amino acids 10–20 were deleted in the TM1 mutant, using the primer 5′-GGGCCGTTGGGGGTGCAGGCCCGGCGGCGCCTCTGAGATCACCT-3′, and amino acids 193–203 were mutated in TM2, using the primer 5′-GCCTATTGGTCAGTAGGAGAACAGGTATTTCTTTTGAAAAGC-3′. Membrane fractionation HEK293-MCT cells were transfected with appropriate plasmids. After 24 h transfection, the cells were treated as directed in results and then scraped into 300 μl of membrane buffer (20 mM Tris, pH 7.5/10 mM MgCl 2 /1 mM EDTA/250 μM sucrose/200 μM phenylmethanesulfonylfluoride). The cells were lysed using 30 strokes of a Dounce homogenizer and spun at 100,000 g for 1 h at 4 °C. The supernatant (cytosolic fraction) was removed to a fresh tube, and the pellet (membrane fraction) was resuspended in 50 μl of sample buffer (50 mM Tris Cl, pH 6.8/10% glycerol (vol/vol)/2% SDS (wt/vol)/0.1% bromophenol blue (wt/vol)/5% 2-mercaptoethanol). The samples were run on a 12% SDS–PAGE gel. Biochemical protease protection assay HEK293-MCT cells were transfected with TMED7-GFP. After 24 h transfection, the cells were trypsinized, washed twice in Dulbecco's modified Eagle's medium, and three times in Krebs–Henseleit buffer (110 mM potassium acetate, 20 mM HEPES (4-(2-hydroxyethyl)-1-piperazineethanesulfonic acid), 2 mM MgCl 2 ). Whole-cell extracts were prepared from one quarter of the cells, and the remaining three quarters were transferred into three reaction tubes. Cells in the three tubes were permeabilized in Krebs–Henseleit buffer containing 20 μM digitonin on ice for 10 min. After permeabilization, one tube was spun down at 100,000 g , 4 °C for 30 min. The supernatant (cytosolic) and the pellet (membrane) were separated and boiled in SDS-Laemmli buffer. The other two tubes were incubated with 1 mM trypsin (Sigma) in the absence or presence of 1% (vol/vol) Triton X-100 (Sigma) on ice for 30 min, and then ultracentrifuged. The pellets were boiled in SDS-Laemmli buffer. We ran the samples on SDS–PAGE and performed western blot analysis using the GFP antibody (Santa Cruz). Statistical analysis Significant differences in mRNA expression following stimulation with LPS were determined by an unpaired two-tailed Student's t -test. A P -value <0.05 was considered statistically significant for all tests. Three independent experiments were carried out in each case ( n =3) and the mean and s.d. were utilized in the t -test. How to cite this article: Doyle, S. L. et al . The GOLD domain containing protein TMED7 inhibits TLR4 signalling from the endosome upon LPS stimulation. Nat. Commun. 3:707 doi: 10.1038/ncomms1706 (2012).